miR-23bandmiR-218silencing increase Muscleblind-like expression and alleviate myotonic dystrophy phenotypes in mammalian models Functional depletion of the alternative splicing factors Muscleblind-like (MBNL 1 and 2) is at the basis of the neuromuscular disease myotonic dystrophy type 1 (DM1). We previously showed the efficacy of miRNA downregulation in Drosophila DM1 model. Here, we screen for miRNAs that regulate MBNL1 and MBNL2 in HeLa cells. We thus identify miR-23b and miR-218 , and confirm that they downregulate MBNL proteins in this cell line. Antagonists of miR-23b and miR-218 miRNAs enhance MBNL protein levels and rescue pathogenic missplicing events in DM1 myoblasts. Systemic delivery of these “antagomiRs” similarly boost MBNL expression and improve DM1-like phenotypes, including splicing alterations, histopathology, and myotonia in the HSA LR DM1 model mice. These mammalian data provide evidence for therapeutic blocking of the miRNAs that control Muscleblind-like protein expression in myotonic dystrophy. Myotonic dystrophy type 1 (DM1) is an autosomal dominant rare genetic disease with variable presentation. It typically involves severe neuromuscular symptoms including cardiac conduction defects, myotonia, and progressive muscle weakness and wasting (atrophy). Neuropsychological dysfunction is also a common symptom of DM1 [1] . The cause of DM1 is well known, namely the accumulation of mutant transcripts containing expanded CUG repeats in the 3′UTR of the dystrophia myotonica protein kinase ( DMPK ) gene. CUG repeats form the disease’s hallmark ribonuclear foci. Mutant DMPK RNA triggers toxic gene misregulation events at the level of transcription [2] , translation [3] , [4] , [5] , [6] , gene silencing [7] , [8] , [9] , [10] , alternative splicing, and polyadenylation of subsets of transcripts [11] , [12] , [13] . RNA toxicity stems from enhanced binding of proteins to expanded CUG RNA, which exists as imperfect hairpin structures. The RNA-binding proteins are thus depleted from their normal cellular targets. Chief among these are the Muscleblind-like proteins (MBNL1–3), whose sequestration contributes to DM1 in several ways. MBNL1 controls fetal-to-adult splicing and polyadenylation transitions in muscle and MBNL2 likely has a similar role in the brain [14] , [15] , whereas Mbnl3 deficit results in age-associated pathologies that are also observed in myotonic dystrophy [16] , [17] . No treatment has yet been specifically developed for DM1 despite intensive efforts. Numerous therapeutic approaches have been designed following different approaches [18] , [19] that can be broadly grouped as: (1) specific targeting of the mutant allele or its RNA product, including preventing MBNL protein sequestration using small molecules [20] , [21] , [22] , [23] , transcriptional [24] , [25] and post-transcriptional silencing of DMPK [26] , and (2) target signaling pathways downstream from CUGexp (CUG expansion) expression [27] , [28] . Two strategies have reached human trials: Tideglusib, a small molecule non-ATP-competitive glycogen synthase kinase 3 (GSK-3) inhibitor [4] (clinical trial NCT02858908) and IONIS-DMPKRx, an RNase H1-active ASO (antisense oligonucleotide) that target CUGexp RNA [29] (clinical trial NCT02312011). However, in IONIS-DMPKRx clinical trial, drug levels measured in muscle biopsy confirmed that the amount of target engagement was not enough to exert a desired therapeutic effect [30] . There is ample evidence that MBNL1 and MBNL2 functions are the limiting factors in DM1. Therefore, boosting their expression is a potential therapeutic avenue. Indeed overexpression of MBNL1 could rescue disease-associated RNA missplicing and muscle myotonia in a DM1 mouse model that expresses 250 CTG repeat units from a human skeletal actin promoter (HSA LR ) [31] , [32] . Consistently, compound loss of Muscleblind-like function reproduces cardinal features of DM1 such as reduced lifespan, heart conduction block, severe myotonia, and progressive muscle weakness [33] . MBNL1 overexpression was well-tolerated in skeletal muscle and early and long-term MBNL1 overexpression prevented CUG-induced myotonia, myopathy, and alternative splicing abnormalities in DM1 mice [34] . Targeted expression of MBNL1 can even rescue eye and muscle atrophy phenotypes in Drosophila DM1 models [35] , [36] , [37] . We recently used a Drosophila DM1 model to show that Muscleblind could be upregulated by sequestration of repressive miRNAs to improve splicing, muscle integrity, locomotion, flight, and lifespan [38] . Here, we extend these studies to mammalian disease models and demonstrate that miR-23b and miR-218 are endogenous translational repressors of MBNL1/2 and MBNL2 , respectively. AntagomiRs transfection upregulates MBNL proteins and rescues alternative splicing in normal and DM1 human myoblasts. Furthermore, systemic administration of antagomiRs in the HSA LR mouse model upregulate Muscleblind-like protein in both gastrocnemius and quadriceps muscles and rescue the molecular, cellular, and functional defects of DM1 muscle. Identification of miRNAs that regulate MBNL1 and MBNL2 We approached a detailed description of MBNL1 and MBNL2 regulation by overexpressing miRNAs in HeLa cells using a commercial kit. The study identified 19 and 9 miRNAs that reduced MBNL1 or MBNL2 transcript levels by at least 4-fold, respectively, compared to controls (Supplementary Fig. 1 ). 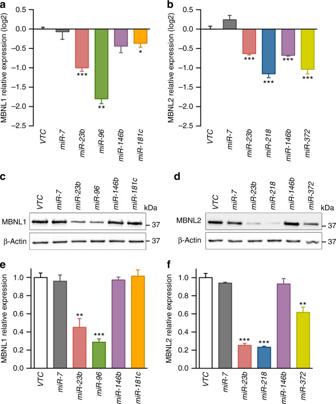Fig. 1 Validation of candidateMBNL1and/orMBNL2regulatory miRNAs. Logarithmic representation on base 2 (log2) of the qRT-PCR quantification ofMBNL1(a) andMBNL2(b) expression relative toGAPDHgene in HeLa cells transfected with the indicatedpCMV-MIRplasmids.c–fRelative protein expression levels of MBNL1 (c,e) and MBNL2 (d,f) in HeLa cells transfected as above. β-ACTIN was the endogenous control. In all cases, emptypCMV-MIR-GFPplasmid (VTC) was used as reference value for relative quantification,miR-37266andmiR-7were used as positive and negative controls, respectively. GFP was used as transfection control. (n= 3). Data are mean ± SEM. *p< 0.05, **p< 0.01, ***p< 0.001 according to Student’sttest We ranked the miRNAs according to likelihood of a direct physical interaction with MBNL1 or MBNL2 3′-UTR sequences (Supplementary Table 1 ). We selected five miRNAs with the best target predictions and also included miR-146b in our validation work because it downregulated MBNL1 the most. Overall, selected miRNAs were: miR-96 and miR-181c as candidate direct repressors of MBNL1 ; miR-218 and miR-372 as candidate repressors of MBNL2 , and miR-146b and miR-23b as potential regulators of both. In validation experiments, HeLa cells were transfected with the corresponding miRNA precursor sequences cloned into the pCMV-MIR-GFP vector. All candidate miRNAs confirmed the expected reduction in endogenous MBNL1 and/or MBNL2 mRNA levels (Fig. 1a, b ), except for miR-146b that only significantly reduced MBNL2 expression. Next, we used western blot quantification to confirm the Muscleblind-like protein downregulation by miRNAs (Fig. 1c–f ). All mRNA reductions were thus confirmed at the protein level except for miR-181c on MBNL1 translation and miR-146b , which failed to repress both MBNL1 and MBNL2. Taken together, these results identified miR-96 , miR-23b , and miR-218 as new miRNAs that repress MBNL1 and/or MBNL2 expression both at the mRNA stability and protein levels. Fig. 1 Validation of candidate MBNL1 and/or MBNL2 regulatory miRNAs. Logarithmic representation on base 2 (log2) of the qRT-PCR quantification of MBNL1 ( a ) and MBNL2 ( b ) expression relative to GAPDH gene in HeLa cells transfected with the indicated pCMV-MIR plasmids. c – f Relative protein expression levels of MBNL1 ( c , e ) and MBNL2 ( d , f ) in HeLa cells transfected as above. β-ACTIN was the endogenous control. In all cases, empty pCMV-MIR-GFP plasmid (VTC) was used as reference value for relative quantification, miR-372 [66] and miR-7 were used as positive and negative controls, respectively. GFP was used as transfection control. ( n = 3). Data are mean ± SEM. * p < 0.05, ** p < 0.01, *** p < 0.001 according to Student’s t test Full size image Mapping of miRNA–mRNA binding sites in the 3′UTR of MBNL1 /2 miRNAs generally act as post-transcriptional repressors by recognizing specific sequences in the 3′-UTR of target mRNAs [39] . To test if our three candidate miRNAs directly bind to the trailer regions of MBNL1 and MBNL2 , as predicted by miRanda [40] and TargetScan [41] (Fig. 2a, e ), we performed reporter assays in HeLa cells. The 3′-UTR of each gene was fused to the Gaussian luciferase reporter (Gluc) so that any functional interaction of a regulatory miRNA and the reporter construct will reduce luminescence measurements. Cotransfection of miRNA target gene luciferase reporter constructs and miRNA plasmids in HeLa cells confirmed a significant decrease in the luciferase luminescence for all tested miRNAs (Fig. 2b, f ). Fig. 2 Confirmation of miRNA binding to MBNL1 and MBNL2 3′UTRs. a , e Scale representation of MBNL1 ( a ) and MBNL2 ( e ) 3′ UTRs and predicted miRNA binding sites according to miRanda and TargetScan algorithms. MBNL1 ( b – d ) and MBNL2 ( f – h ) 3′ UTR luciferase reporter assays of HeLa cells co-transfected with wild-type ( b , f ) or mutated ( c , d , g , h ) versions of 3′ UTR fused to Gaussia luciferase and miRNA plasmids ( n = 4). miR-7 was used as a negative control. Wild-type (WT) reporter plasmids had the natural sequence of the miRNA binding sites, mutated (MUT) constructs lacked a candidate miRNA seed region recognition site and the perfect match (PM) versions had the miRNA binding site replaced by the full complementary sequence. ** p < 0.01, *** p < 0.001 according to Student’s t test. Data are mean ± SEM Full size image miRNA–mRNA interaction strongly depends on the perfect complementarity between the target mRNA and the miRNA seed region at positions 2–8 [39] . Next, we investigated direct binding of miRNAs to single or multiple MBNL 3′-UTR sequences. We made a series of miRNA target gene luciferase reporter plasmids with natural (WT), perfectly matched (PM), or absent (MUT) miRNA recognition sites. In these assays, WT versions of the 3′-UTR of MBNL1 and MBNL2 significantly reduced expression of the Gluc reporter when co-transfected with miR-23b or miR-96 ( MBNL1 ; Fig. 2c, d ), and miR-23b or miR-218 ( MBNL2 ; Fig. 2g, h ). In comparison, cotransfection with the corresponding mutant versions always abrogated the repressive effect of the miRNAs whereas PM versions had lower luciferase than WT constructs. Strikingly, deletion of any of the three miR-218 recognition sites in MBNL2 alleviated full repression of the Gluc reporter. Overall, we conclude that miR-96 , miR-218 , and miR-23b , directly regulate MBNL1 , MBNL2 , or both genes, respectively. miR-23b and miR-218 antagomiRs stabilize MBNL transcripts DM1 pathology depends on Muscleblind-like protein expression in muscle. A pre-requisite for the hypothesis that miRNAs fine-tune MBNL1 and/or MBNL2 translation in muscle was that our candidate miRNAs were expressed there. We therefore measured levels of miR-96 , miR-23b , and miR-218 in muscle by qPCR. miR-23b and miR-218 were highly expressed in cultured human DM1 myoblasts and muscle biopsies, whereas miR-96 was found at negligible levels (Fig. 3a ). To test this potential of miR-23b and miR-218 as therapeutic targets for DM1, we designed antisense oligonucleotides (antagomiRs) that recognize these miRNAs. AntagomiRs are very stable and have cholesterol moieties to enhance their uptake into cells [42] , [43] . First, we characterized their toxicity profiles. The TC10 concentrations (at which at least 90% of cells remained viable) were 654.7 nM for antagomiR-23b and 347 nM for antagomiR-218 (Fig. 3b ). Fig. 3 AntagomiR-23b and -218 stabilize MBNL transcripts and rescue alternative splicing defects in DM1 myoblasts. a Real-time PCR quantification of miR-96 , miR-23b , and miR-218 expression in myoblasts and muscle biopsies from DM1 patients. U1 and U6 snRNAs were used as reference genes. b Cell growth inhibition assay by MTS method. Human normal myoblasts were transfected with increasing concentrations of antagomiRs against miR-23b and miR-218 ( n = 4). TC10 was obtained using the least squares non-linear regression model. c , d qRT-PCR quantification of MBNL1 ( c ) and MBNL2 ( d ) expression relative to GAPDH and ACTB genes in human DM1 myoblasts transfected with the indicated antagomiRs or scrambled control antagomiR (sc). e Semiquantitative RT-PCR analyses of splicing events altered in BIN1 (exon 11), ATP2A1 (exon 22), cTNT (exon 5), INR (exon 11), and PKM isoforms in DM1 cells. GAPDH was used as internal control. Inclusion of DLG1 exon 9, which is not altered in DM1, and CAPZB exon 8, which is CELF1-dependent, were used as additional controls. f , h miRNA real-time PCR determination of available miR-23b ( f ) or miR-218 ( h ) in DM1 myoblasts 96 h after transfection with 50 nM of antagomiR-23b or 200 nM of antagomiR-218. U1 and U6 snRNAs were used as reference genes in f and h . g , i qRT-PCR analyses of MBNL1 ( g ) and MBNL2 ( i ) expression relative to GAPDH and ACTB genes in human myoblasts 96 h after transfection with 50 nM of antagomiR-23b or 200 nM of antagomiR-218. ( n = 3). Data are mean ± SEM. * p < 0.05, ** p < 0.01, *** p < 0.001 according to Student’s t test Full size image Visual confirmation of cell uptake was obtained with Cy3-labeled versions of antagomiRs at concentrations ranging 50–100 nM, but not at 10 nM (Supplementary Fig. 2 ). Having established the effective and non-toxic range for the antagomiRs, we tested the ability of antagomiR-23b and -218 to block their corresponding miRNA at concentrations at which cell uptake was confirmed (>50 nM), but well below TC10. DM1 myoblasts were transfected with antagonists and the mRNA levels of MBNL1 and MBNL2 were measured 48 and 96 h later. MBNL1 and MBNL2 transcripts in cells treated with antagomiR-218 increased in a dose-dependent manner at both time points and reached approximately 50% higher levels than in scramble control-treated DM1 cells (Fig. 3c, d ). Of note, since silencing of miR-218 enhanced MBNL1 transcripts but did not bind to the MBNL1 3′-UTR reporter constructs (Supplementary Fig. 3 ) regulation by this miRNA might be indirect or dependent on sequences outside the 3′-UTR. In sharp contrast to miR-218 blockers, the lower the concentration of antagomiR-23b the higher the increase in MBNL levels. MBNL1 transcripts doubled in DM1 cells 96 h post-transfection with 50 nM of antagomiR-23b. Assuming a typical bell-shaped dose–response, these results suggested that working concentration for antagomiR-23b is 50 nM, or lower, and 200 nM or higher for antagomiR-218 (Fig. 3c, d ). Importantly, levels of miR-218 were not altered in cells treated with antagomiR-23b, suggesting a specific effect of the antagomiR on its target. miR-23 family includes miR-23a and miR-23b , which are transcribed from different chromosomes, have identical seed sequences, and differ by only one nucleotide on their 3′ ends. As expected, antagomiR-23b also reduced the levels of miRNA-23a in the cells (Supplementary Fig. 4a, b ). In summary, we have confirmed the ability of miR-23b and miR-218 antagonists to enter DM1 cells and enhance MBNL1 and MBNL2 mRNA levels, at concentrations well below their toxicity threshold. miR-23b and miR-218 silencing rescues defects in DM1 cells The best-known molecular alteration in DM1 is missplicing of defined subsets of muscle transcripts. To test whether higher amounts of MBNL1 and MBNL2 mRNA translate into rescue of the Muscleblind-dependent splicing events, we transfected DM1 cells using the optimal conditions determined above and verified improvement of missplicing events including Bridging integrator 1 ( BIN1 ) [44] , ATPase sarcoplasmic/endoplasmic reticulum Ca 2+ transporting 1 ( ATP2A1) [45] , Insulin receptor ( INSR) [46] , [47] , and Piruvate kinase M ( PKM ) [48] . Exon inclusion (Percentage Spliced In; PSI) was significantly rescued for all four transcripts 96 h post-transfection (Fig. 3e ; Supplementary Fig. 5 ) upon miR-23b or miR-218 silencing (Fig. 3f, h ). Similarly, BIN1 , ATP2A1 , and PKM splicing, but not INSR , was also rescued 48 h after antagomiR transfection (Supplementary Figs. 5 and 6 ). In contrast, increased levels of MBNL1 and MBNL2 in DM1 myoblasts did not significantly change the aberrant inclusion of exon 5 in the Cardiac troponin T ( cTNT ) [46] transcripts under any of the experimental conditions tested. To test the specificity of antagomiRs-23b and -218, we quantified the inclusion of exon 8 of CAPZB , which depends on CUGBP Elav-like protein family member 1 (CELF1) [49] , and observed that it was not rescued by the antagomiRs (Fig. 3e ; Supplementary Figs. 5 and 6 ). Additionally, the regulated inclusion of exon 19 of DLG1 , which is known to be MBNL1 and CELF1 -independent, did not change under any of the experimental conditions, thus discarding global effects on alternative splicing control upon antagomiR treatment (Fig. 3e ; Supplementary Figs. 5 , 6 ). Taken together, these results confirm Muscleblind-specific rescue of alternative splicing defects taking place in DM1 myoblasts as a result of antagomiR-mediated MBNL1 and MBNL2 derepression. AntagomiRs-23b/-218 restore normal MBNL cell distribution Since miRNAs can regulate gene expression at the mRNA stability and translation levels, we sought to determine the effect of antagomiRs on MBNL1 and MBNL2 protein expression. Upon antagomiR treatment, qPCR data confirmed a significant increase in the levels of MBNL1 and MBNL2 mRNA 96 h (Fig. 3g, i ) or 48 h (Supplementary Fig. 6 ) post-transfection. At the protein level, these differences were further enhanced and western blots detected 4–5-fold more MBNL1, and 3–5-fold higher MBNL2 proteins, in DM1 myoblasts after 96 h (Fig. 4a, b, d, e ) and 48 h (Supplementary Fig. 6 ) of antagomiR treatment. Of note, MBNL1 and MBNL2 protein levels remained unaltered in control and DM1 cells mock-transfected or transfected with a scrambled control antagomiR (Supplementary Fig. 7 ). In contrast, CELF1 protein levels remained unchanged upon miR-23b or miR-218 silencing (Fig. 4c, f ; Supplementary Fig. 6 ) and, consistently, CAPZB alternative splicing remained the same. Importantly, this increase was clearly visible by immunofluorescence. Whereas both MBNL1 and MBNL2 were sequestered in ribonuclear foci of DM1 myoblasts (Fig. 4 h, l), antagomiRs-23b and -218 robustly increased the protein expression and restored their distribution in the cytoplasm and in the cell nucleus (Fig. 4 i, j, m, n). The increase of MBNL1 and MBNL2 proteins in the cell nucleus was consistent with the previously shown splicing rescue. Because the relationship between MBNL proteins and CUGexp foci formation is complex, a potential undesirable side effect of boosting MBNL expression was an increase in the number of ribonuclear foci. To specifically test this hypothesis, we quantified foci in antagomiR-treated DM1 fibroblasts and found that remained unaltered (Fig. 4o–r ). Fig. 4 Increase of MBNL1 and MBNL2 upon silencing of miR-23b or miR-218 in human myoblast. a – f Western blot quantification of MBNL1 ( a , d ), MBNL2 ( b , e ), and CELF1 ( c , f ) expression levels in DM1 human myoblast 96 h after transfection with 50 nM of antagomiR-23b, 200 nM of antagomiR-218 or a scrambled control antagomiR (sc). β-ACTIN expression was used as endogenous control ( n = 3). Data are mean ± SEM. ** p < 0.01, *** p < 0.001 in Student’s t test. g – n Representative confocal images of MBNL1 (green) and MBNL2 (red) staining in healthy controls (control cells) and DM1 human myoblast 96 h after transfection with antagomiRs against miR-23b (50 nM) or miR-218 (200 nM) and a scrambled control antagomiR (DM1 cells). Nuclei were counterstained with DAPI (blue). In DM1 cells, endogenous MBNL1 ( h ) and MBNL2 ( l ) were in nuclear aggregates (green and red puncta) and the total amount of both was reduced compared to control cells ( g ) and ( k ), respectively. In contrast, DM1 cells treated with antagomiRs against miR-23b or miR-218 showed a robust increase in cytoplasmic and nuclear MBNL1 ( i , j ) and MBNL2 ( m , n ) levels compared to DM1 cells. b – q Representative fluorescence of FISH images showing (CUG)n RNA foci (red) in DM1 human fibroblasts transfected with antagomiRs against miR-23b (50 nM) or miR-218 (200 nM) and a scrambled control antagomiR. Nuclei were counterstained with Hoechst (blue). AntagomiRs did not significant change the number of ribonuclear foci in DM1 fibroblasts ( r ). Scale bar = 20 μm Full size image miR-23b and miR-218 are expressed in tissues relevant to DM1 To obtain a broader view of the expression pattern and relative expression of these miRNAs, we turned to mouse tissue samples, using the reference FVB strain. We analyzed muscle (quadriceps, gastrocnemius), whole heart, and central nervous system (forebrain, cerebellum, hippocampus). All samples had robust expression of miR-23b and miR-218 , whereas miR-96 was again almost undetectable except in cerebellum (Fig. 5a ). miR-218 was expressed up to 80 times higher in brain tissues than in muscle-derived samples. miR-23b and miR-218 are therefore strongly expressed in the tissues that are highly relevant to DM1 pathology (skeletal muscle, heart, brain) where they likely repress MBNL1 and/or MBNL2 translation. Since levels of MBNL proteins are limiting in DM1, miR-23b and miR-218 may be contributing to the disease phenotypes and can be regarded as potential therapeutic targets. Fig. 5 Subcutaneous injection of antagomiR-23b or antagomiR-218 in HSA LR mice reduced target miRNA levels and increased Mbnl1 and Mbnl2 without affecting levels of Celf1. a qPCR quantification of miR-96 , miR-23b , and miR-218 expression levels in forebrain (fb), cerebellum (cb), hippocampus (hp), heart (ht), and quadriceps (qd) and gastrocnemius (gt) muscles ( n = 3). Average expression levels of U1 and U6 were used for normalization. b – e Immunodetection of Cy3-labeled antagomiRs in gastrocnemius ( b , d ) and quadriceps ( c , e ) cryosections of HSA LR treated mice ( n = 1). Myonuclei were counterstained with DAPI (blue). Scale bar = 50 μm. f – g Quantification of miR-23b and miR-218 in gt and qd muscles of untreated mice (PBS, gray bars) or treated with antagomiR-23b (pink bars) or antagomiR-218 (blue bars). Relative values (to average of U1 and U6 expression) were further normalized to the levels in untreated mice. h, i Real-time PCR quantification of Mbnl1 and Mbnl2 transcript levels in gt and qd muscles. Expression levels relative to the endogenous Gapdh were normalized to the levels in untreated mice. j – o Western blotting analysis of Mbnl1 ( j , m ), Mbnl2 ( k , n ), and Celf1 ( l , o ) proteins in mouse gt and qd muscles. Representative blots used for quantification in ( m – o ) are shown in ( j – l ). The data were analyzed by unpaired Student’s t test compared to untreated HSA LR mice. Data are mean ± SEM. * p < 0.05, ** p < 0.01, *** p < 0.001; HSA LR PBS ( n = 10 in f – o ), HSA LR antagomiR-23b ( n = 9, in f – o ). HSA LR antagomiR-218 ( n = 9, in f – o ) Full size image AntagomiRs increase Mbnl expression in HSA LR mouse muscle Next, we investigated the activity of antagomiR-23b and -218 in the HSA LR mouse DM1 model [31] . First, we evaluated the ability of antagomiRs to reach skeletal muscle. Cy3-labeled versions of the antagomiRs were administered to a 4-month-old HSA LR mouse by a single subcutaneous injection. Four days post-injection, hind limb gastrocnemius and quadriceps muscles were processed to detect the labeled oligonucleotide. We observed the antagomiRs by anti-Cy3 immunofluorescence in a strong punctate pattern in nuclei and membrane of both muscles. The antagomiRs were also diffusely present throughout the cells (Fig. 5b–e ). These data demonstrate that antagomiR oligonucleotides that block miR-23b or miR-218 can reach the skeletal muscles of a DM1 mouse model. We decided to inject unlabeled antagomiRs to nine additional DM1 animals, in three consecutive injections (12 h intervals) to a final dose of 12.5 mg kg −1 . The controls were injected with PBS1x ( n = 10) or scrambled antagomiR ( n = 5). Four days after the first injection, animals were sacrificed and quadriceps and gastrocnemius were obtained for histological and molecular analysis. We confirmed that miR-23b and miR-218 were strongly silenced by their complementary antagomiRs. miR-23b was reduced to 30–40% and miR-218 to 50% of the levels measured in the untreated HSA LR mice (Fig. 5f, g ). As a result of miRNAs reduction, Mbnl1 and Mbnl2 increased at the transcript and protein levels in both muscle types (Fig. 5h, i, j, k, m, n ). Importantly, levels of Celf1 protein were not altered by either treatment (Fig. 5l, o ). In mice injected with PBS or with scrambled oligo as control, target microRNAs and the Mbnl1 and Mbnl2 transcript levels were indistinguishable (Supplementary Fig. 8a–d ). AntagomiRs rescue missplicing of muscle transcripts in mice Given the robust increase in Mbnl1 and 2 in treated gastrocnemius and quadriceps muscles, we sought to confirm a rescue of Mbnl-dependent splicing events Atp2a1, Chloride channel protein 1 (Clcn1) , and Nuclear factor 1 X-type ( Nfix) in HSA LR mice (Fig. 6a, b ; Supplementary Fig. 9 ). AntagomiR administration ameliorated aberrant exon choices for Atp2a1 (exon 22) and Nfix (exon 7), and increased Clcn1 exon 7a PSI in gastrocnemius but not in quadriceps of HSA LR mice. To test the specificity of antagomiRs-23b and -218 on MBNL regulation, we quantified the inclusion of exon 8 of Capzb , Exon 21 of Ank2 , and exon 3 of Mfn2 , which depend on Celf1 [49] , [50] , and observed that they were not altered by treatment with antagomiRs. Fig. 6 Systemic delivery of antagomiRs improved missplicing of Mbnl-dependent transcripts, myotonia, and muscle histopathology in HSA LR mice. a , b RT-PCR analyses of the splicing of Atp2a1 exon 22, Clcn1 exon 7a, Nfix exon 7, Capzb exon 8, Ank2 exon 21, and Mnf2 exon 3 in gastrocnemius (gt) ( a ) and quadriceps (qd) ( b ) muscles. Gadph values were used for normalization in the quantification of the exon inclusion in Supplementary Figs. 9 and 11 . c Electromyographic myotonia grade in antagomiR (pink and blue bars) or PBS-treated (gray bars) HSA LR mice before (bi) and 4 days after injection (ai). Data are mean ± SEM. d Quantification of the percentage of muscle fibers with central nuclei in gt and qd muscles of control FVB (white bar), and PBS (gray bar) or antagomiR-treated (pink and blue bars) HSA LR mice. e – h Representative hematoxylin and eosin staining of gt muscles from all four groups of mice. Arrows point to examples of centrally located nuclei in muscle fibers. Scale bar = 50 μm. The data were analyzed by unpaired Student’s t test compared to untreated HSA LR mice. Data are media ± SEM. * p < 0.05; FVB ( n = 3), HSA LR PBS ( n = 5), HSA LR antagomiR-23b ( n = 4) and HSA LR antagomiR-218 ( n = 4) Full size image In a routine test of transgene expression of HSA LR mice, we discovered that CUG expression levels varied up to 0.5-fold among animals and that variation positively correlates with aberrant inclusion of alternative exons in gastrocnemius and quadriceps (Supplementary Fig. 10 ). To note Atp2a1 exon 22 inclusion was bimodal. Two out of 10 mice that expressed low levels of transgene included exon 22 to levels significantly higher (closer to normal) than the rest of HSA LR mice and were therefore excluded from the analysis (Supplementary Figs. 10 and 11 ). These data suggest that the lower the expression of CUG repeat RNA in muscles the less missplicing there is. In contrast, in the antagomiR-treated HSA LR muscle samples splicing defects correlated with Mbnl mRNA levels, instead of repeat expression, which supported a causal role of these proteins in the rescue of the splicing events (Supplementary Fig. 10 ). Despite the intrinsic variability of the model, we conclude that both antagomiRs achieved similar levels of rescue in all gastrocnemius-missplicing events. However, antagomiR-23b rescued Nfix splicing to a greater extent than antagomiR-218 in quadriceps, which correlated with the lower upregulation of Mbnl1 and 2 protein levels achieved by antagomiR-218 in this muscle. Consistent with the unchanged levels of Celf1 protein in the muscles of treated HSA LR mice, inclusion percentage of Celf1 -dependent splicing events in gastrocnemius and quadriceps of treated and control mice was very similar (Fig. 6a, b and Supplementary Fig. 9 ). Importantly, the Mbnl1 and 2 protein levels and the splicing patterns of Mbnl- or Celf1-dependent events in mice injected with PBS or with scrambled oligo, as control, were indistinguishable (Supplementary Fig. 8e–i ). These results indicate that systemic delivery of antagomiRs was able to rescue muscle missplicing in vivo in a DM1 mouse model. AntagomiRs improve muscle histopathology and reduce myotonia Defective transitions of fetal to adult alternative splicing patterns have been proposed to originate DM1 muscle phenotypes [51] . In HSA LR DM1 model mice, alterations in ionic currents cause repetitive action potentials, or myotonia, that can be quantified by electromyography. Before treatment, all DM1 mice had grade 3 or 4 myotonia, i.e., abundant repetitive discharges with the vast majority of electrode insertions. Four days after, antagomiRs reduced myotonia to grade 2 (myotonic discharge in >50% of insertions) or grade 1 (occasional myotonic discharge) in 55% of the mice treated with antagomiR-218, and in 50% of the mice treated with antagomiR-23b, respectively (Fig. 6c ). A typical histological hallmark of DM1 and HSA LR mouse muscle fibers is a central location of nuclei, which results from myopathic muscle attempting to regenerate [5] . Both antagomiRs caused decentralization of nuclei in both gastrocnemius and quadriceps muscles (Fig. 6d–h ). In contrast, myotonia levels and number of central nuclei remained unaltered in mice treated with the scrambled antagomiR (Supplementary Fig. 8j–m ). Taken together, these results validate the potential of antagomiR-23b and -218 as a drug that suppresses CUG-repeat RNA-induced myopathy in mammals. AntagomiR long-term treatment rescue functional phenotypes In order to assess the long-term effects of the antagomiR treatments, we studied characteristic molecular and functional alterations in the HSA LR mice in groups of mice treated with the same dose and posology as before but sacrificed 6 weeks after the antagomiR injections. The levels of miR-23b and miR-218 in these mice were still significantly reduced 6 weeks after the initiation of the experiment, but the reduction was less pronounced than in the short-term treatment. In general, the reduction of target miRNAs was not enough to maintain the increased Mbnl transcript levels, as only Mbnl1 transcripts in quadriceps were significantly augmented 6 weeks after injection (Fig. 7a–d ). Myotonia grade measured before injection (bi), in the halfway point (hp, 3 weeks after the injection) and in the final point (fp, before sacrifice) showed a clear tendency to decrease with time (Fig. 7e ), and forelimb muscle force measured in the final point and normalized to body weight, increased in both treatments although the difference was only significant for antagomiR-218 (Fig. 7f ). Fig. 7 Muscle function is improved in HSA LR mice 6 weeks after injection of antagomiRs. a , b qRT-PCR quantification of Mbnl1 and Mbnl2 transcript levels in gt and qd muscles of untreated mice (PBS, gray bars) or treated with antagomiR-23b (pink bars) or antagomiR-218 (blue bars). c , d Real-time PCR quantification of miR-23b and miR-218 . e Electromyographic myotonia grade in antagomiR (pink and blue bars) or PBS-treated (gray bars) HSA LR mice before (bi), in the halfway-point (hp) and 6 weeks after injection (final point, fp). f Forelimb grip strength of mice treated with antagomiRs measured before injection (bi) and 6 weeks after injection (fp). The grip force was normalized with the body weight of each mouse. The data were analyzed by unpaired Student’s t test compared to HSA LR mice treated with the vehicle PBS. Data are mean ± SEM. * p < 0.05, *** p < 0.001; FVB ( n = 5), HSA LR PBS ( n = 6), HSA LR antagomiR-23b ( n = 5) and HSA LR antagomiR-218 ( n = 5) Full size image Importantly, visual necropsy and biochemical blood parameters measured of the mice before sacrifice support a non-deleterious effect of the treatment with the antagomiRs, even after 6 weeks (Supplementary Data 2 ). The only parameters altered in these analyses were total bilirubin, which was decreased in all treated animals, potentially reflecting an increase in liver metabolic rate, and monocyte number, which increased also in all treated animals, suggesting activation of the immune system. Given that these two parameters were also altered in the scrambled-treated mice, the alterations might be caused by the oligo chemistry instead of specific microRNA inhibition. A largely unexplored therapeutic strategy for DM1 is therapeutic gene modulation (TGM), which pursues to raise or lower the expression of a given gene to alleviate a pathological condition. Examples of TGM are inhibition of CD44 in metastatic prostate cancer [52] , or the pharmacological enhancement of utrophin expression to compensate lack of dystrophin in Duchenne Muscular Dystrophy [53] . Previous attempts to raise the critically low levels of Muscleblind in DM1 involved epigenetic upregulation of endogenous MBNL1 [54] or derepression of muscleblind by sponge-mediated silencing of miRNAs in a Drosophila DM1 model [38] . Oligonucleotide-based modulation of miRNA activity has prompted great attention because of its efficacy in animal models of disease and the development of specialized chemistries [52] , [55] , [56] . In this study, we identified miR-23b and miR-218 as inhibitors of MBNL1 and MBNL2 translation, and show that complementary antagomiRs robustly silence their target miRNAs in patient-derived myoblasts and HSA LR mouse model. We found that antagomiRs are effective at doses lower than those previously reported in muscle [43] , [57] , [58] . By inhibiting miR-23b and miR-218 in mouse muscle, we were able to upregulate MBNL1 and MBNL2 protein levels by approximately over 2-fold and 4-fold, respectively, without affecting CELF1 levels. Importantly, MBNL protein overexpression was previously shown to be well-tolerated in mouse models [34] . Accordingly, in our study, upregulation of MBNL proteins through miR-23b or miR-218 silencing was not harmful, as mice showed no detrimental phenotype 6 weeks after the treatment. Similarly, miR-23b silencing in the heart of an inducible DM1 mice model caused no overt phenotype, despite producing CELF1 overexpression [59] . This data supports the safety of our therapeutic approach in DM. Although different effects of antagomiR-23b on CELF1 levels are reported in these two studies, antagomiR dose used or tissue-specific effects might explain this controversy. Given the tissue-specific expression of microRNAs, their targeting in TGM is also advantageous because it regulates genes only in the places where the regulator miRNAs are expressed, and the intensity of the upregulation will depend on the degree of repression by that microRNA. Several previous studies have reported that phenotypes of HSA LR model mice are intrinsically variable [4] , [60] . This was suggested to stem from somatic instability of CUG repeats [4] , but we found that the levels of expression of the HSA LR transgene and the magnitude of missplicings have a strong positive correlation. Indeed, for some splice events such as Atp2a1 , small changes in transgene expression translated into big changes in exon inclusion. We suggest that the quantification of the transgene expression is an important step in order to identify outliers. It is well known that sequestration of MBNLs and activation of CELF1 block the developmental change from fetal to adult RNA transcripts in DM1 muscle. We demonstrate that upregulated MBNL1 and MBNL2 was sufficient to rescue several Muscleblind-dependent, but not the CELF1-dependent splice events, in DM1 myoblasts and HSA LR DM1 model mice. Interestingly, a mere 2-fold increase of Mbnl2 (and a marginal increase in Mbnl1) protein in quadriceps was sufficient to strongly rescue Nfix missplicing. Thus, we found that a relatively small upregulation of the MBNL proteins can have a profound impact on DM1 phenotypes not only at the level of missplicing but also at histopathology (central nuclei) and functional (myotonia and muscle strength) levels. Overall our study highlights the use of oligonucleotide drugs to specifically de-repress the expression of the MBNL1 and MBNL2 genes as therapeutic approach for DM1. Cell culture HeLa cells were obtained from Dr. Francisco Palau (Sant Joan de Deu Hospital, Spain) and were grown in Dulbecco’s Modified Eagle’s Medium (DMEM) with 1 g L −1 glucose, 1% penicillin and streptomycin (P/S), and 10% fetal bovine serum (FBS; Sigma). Unaffected (control) and patient-derived cells (DM1 cells carrying 1300 CTG repeats quantified in the blood cells) [61] were kindly provided by Dr. Furling (Institute of Myology, Paris). Fibroblast cells were grown in DMEM with 4.5 g L −1 glucose, 1% P/S, and 10% FBS (Sigma). To transdifferentiate fibroblasts into myoblasts by inducing MyoD expression, the cells were plated in muscle differentiation medium (MDM) containing DMEM with 4.5 g L −1 glucose, 1% P/S, 2% horse serum, 1% apo-transferrin (10 mg ml −1 ), 0.1% insulin (10 mg ml −1 ), and 0.02% doxycycline (10 mg ml −1 ). In all cases, the cells were grown at 37 °C in a humidified atmosphere containing 5% CO 2 . MicroRNA profiling To search for miRNAs that regulate MBNL1 and MBNL2 in HeLa cells, the SureFIND Cancer miRNA Transcriptome PCR Array (Qiagen) was used according to the manufacturer’s instructions. Briefly, a multiplex quantitative real-time PCR (qRT-PCR) assay was set up using the QuantiFast Probe PCR Kit reagent with TaqMan probes gene expression assays for human MBNL1 and MBNL2 (FAM-labeled probe) and GAPDH (MAX-labeled probe; Qiagen). qRT-PCR was performed using a StepOnePlus real-time thermal cycler and the results were analyzed using Excel-based data-analysis software provided with the SureFIND miRNA Transcriptome PCR Array. MBNL1 and MBNL2 gene expression was normalized to GAPDH. Computational prediction of miRNA targets in MBNL1/2 3′ UTRs Information about the predicted miRNA binding to MBNL1 and MBNL2 was obtained from miRecords [62] and miRDIP [63] databases. These databases integrate nine different programs (microT, MiRanda, MirTar2_V4.0, Mir Target2, Pic Tar, PITA, RNA hybrid, RNA 22, and TargetScan) that predict miRNA targets. A miRNA was considered as a candidate regulator if it was predicted by at least eight of these prediction algorithms. TargetScan (release 6.2) and MiRanda (release August 2010) were used to design the 3′UTR reporter assay, which allows analysis of the miRNA–mRNA binding sites. AntagomiRs Cy3-labeled and non-labeled oligonucleotides were synthesized by Creative Biogene. The antagomiR sequences were as follows: 5′‐mG*mG*mUmAmAmUmCmCmCmUmGmGmCmAmAmUmGmU*mG*mA*mU*‐3′-chol (antagomiR-23b) 5′‐mA*mC*mAmUmGmGmUmUmAmGmAmUmCmAmAmGmCmA*mC*mA*mA*-3′-chol (antagomiR‐218) 5′‐mC*mA*mGmUmAmCmUmUmUmUmGmUmGmUmA*mC*mA*mA*‐3′-chol (scramble control, SC) where m denotes 2′- O -methyl-modified phosphoramidites, * denotes phosphorothioate linkages, and chol denotes cholesterol groups. Cy3‐labeled oligonucleotides were used to visualize the distribution of the compound in cells and mouse tissues. Cell transfection HeLa cells and human myoblasts were transfected using X-tremeGENE™ HP (Roche) according to the manufacturer’s protocols. For the miRNA overexpression assay, HeLa cells were seeded in 6-well plates at approximately 80% confluence and transfected with 1 µg of miRNA precursor sequences cloned into the pCMV-MIR-GFP vector (OriGene). At 48 h post-transfection, the cells were harvested for the qRT-PCR and western blot analyses. For the reporter assays, the cells were seeded in 24-well plates at approximately 80% confluence and transfected with MBNL1 and MBNL2 3′UTR luciferase constructs cloned into a pEZX-MT05-Gluc vector (GeneCopoeia). For each transfection, 500 ng of the appropriate reporter construct and 500 ng of the appropriate miRNA plasmids (OriGene) were used. In the case of miR-23b , miR-96 , and miR-218 , three types of constructs were tested, wild-type (WT), perfect match (PM), and constructs with a deletion in the seed region (MUT) predicted to disrupt binding. Both PM and MUT were provided by GeneCopoeia (see Supplementary Data 1 ). The supernatant was collected 48 h after transfection and the reporter activity was assayed. Control fibroblasts were seeded into 96-well plates (1 × 10 5 cells per well), transfected with different antagomiR concentrations (from 1 nM to 1 µM) and transdifferentiated into myoblasts for 96 h in MDM medium; to analyze the toxicity. As a control to test the transfection levels, the Cy3-antagomiR was transfected in separate experiments under the same conditions. For the RT-PCR, qRT-PCR, and Western blot assays, control and DM1 fibroblasts were plated into petri dishes (1 × 10 6 cells per well), transfected with the appropriate antagomiR, and then differentiated for 48 or 96 h. Additionally, for the RT-PCR, control fibroblasts were plated into petri dishes (1 × 10 6 cells per well), transfected with the scrambled control antagomiR, and then differentiated for 48 or 96 h. Finally, for the immunofluorescence and foci assay, fibroblasts were seeded into 24-well plates (3 × 10 5 cells per well), transfected with the relevant antagomiRs, and transdifferentiated into myoblasts for 96 h. Transgenic mice and antagomiR administration Mouse handling and experimental procedures conformed to the European law regarding laboratory animal care and experimentation (2003/65/CE) and were approved by Conselleria de Agricultura, Generalitat Valenciana (Uso de bloqueadores de miRNAS como terapia potencial en distrofia miotónica, reference number 2016/VSC/PEA/00155). Homozygous transgenic HSA LR (line 20 b) mice [31] were provided by Prof. C. Thornton (University of Rochester Medical Center, Rochester, NY, USA) and mice with the corresponding genetic background (FVB) were used as controls. Age-matched HSA LR (<5 months old) male mice received three subcutaneous injections of 100 µl of 1× PBS (vehicle) ( n = 10) or antagomiR (antagomiR-23b n = 9, antagomiR-218 n = 9, and antagomiR-SC n = 5) delivered to the interscapular area every 12 h. The overall quantity of antagomiR finally administered divided among the three injections was 12.5 mg kg −1 . For the long-term treatment, the same injection procedure was used in mice of 3.5 months in age (PBS, antagomiR-23b, antagomiR-218 and antagomiR-SC n = 5). Four days and 6 weeks after the first injection, the mice were sacrificed and the tissues of interest were harvested and divided into two samples each. One part was frozen in liquid nitrogen for the molecular analyses, and the other was fixed in 4% paraformaldehyde (PFA) and cryoprotected in 30% sucrose before histological processing. Cy3-labeled antagomiRs were administered in a single subcutaneous injection of 10 mg kg −1 . RNA extraction, RT-PCR, and qRT-PCR Total RNA from HeLa cells, human myoblasts, and murine muscle tissues was isolated using the miRNeasy Mini Kit (Qiagen; Valencia, CA) according to the manufacturer’s instructions. One microgram of RNA was digested with DNase I (Invitrogen) and reverse-transcribed with SuperScript II (Invitrogen) using random hexanucleotides; 20 ng of cDNA was used in a standard PCR reaction with GoTaq polymerase (Promega). Specific primers were used to analyze the alternative splicing of BIN1 , ATP2A1 , INR , PKM , cTNT , CAPZB , and DLG1 in control and DM1 human myoblasts, and Atp2a1 , Clcn1 , Nfix , Capzb [54] , Ank2, and Mfn2 in mouse samples (quadriceps and gastrocnemius). GAPDH and Gapdh were used as endogenous controls using 0.2 ng of cDNA. In the case of PKM , PCR products were digested with Pst I (Thermo Scientific™). PCR products were separated on a 2% agarose gel and quantified using ImageJ software (NIH). 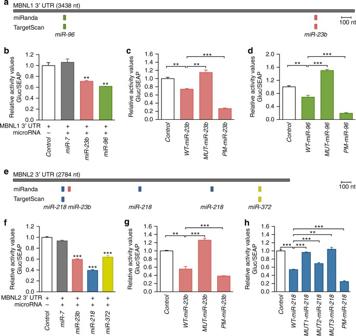Fig. 2 Confirmation of miRNA binding toMBNL1andMBNL23′UTRs.a,eScale representation ofMBNL1(a) andMBNL2(e) 3′ UTRs and predicted miRNA binding sites according to miRanda and TargetScan algorithms.MBNL1(b–d) andMBNL2(f–h) 3′ UTR luciferase reporter assays of HeLa cells co-transfected with wild-type (b,f) or mutated (c,d,g,h) versions of 3′ UTR fused to Gaussia luciferase and miRNA plasmids (n= 4).miR-7was used as a negative control. Wild-type (WT) reporter plasmids had the natural sequence of the miRNA binding sites, mutated (MUT) constructs lacked a candidate miRNA seed region recognition site and the perfect match (PM) versions had the miRNA binding site replaced by the full complementary sequence. **p< 0.01, ***p< 0.001 according to Student’sttest. Data are mean ± SEM The primer sequences and exons analyzed are provided in Supplementary Table 2 . We used 1 ng of HeLa, human myoblast, or mouse tissue cDNA as a template for multiplex qRT-PCR using the QuantiFast Probe PCR Kit reagent. Commercial TaqMan probes (Qiagen) were used to detect human ( MBNL1 and MBNL2 ) or mouse ( Mbnl1 and Mbnl2 ; FAM-labeled probes) and reference ( GAPDH ; MAX-labeled probe) genes. Results from myoblasts were normalized to GAPDH and ACTB (TAMRA-labeled probe; Integrated DNA Technologies) whereas the mouse results were normalized to Gapdh only. HSA transgene expression levels were determined by qRT-PCR as described previously [64] . miRNA expression in human DM1 myoblasts, muscle biopsies, and murine tissues (muscle, heart, and central nervous system) was quantified using specific miRCURY™-locked nucleic acid microRNA PCR primers (Exiqon) according to the manufacturer’s instructions. Relative gene expression was normalized to U1 or U6 snRNA. Expression levels were measured using an Applied Biosystems StepOnePlus Real Time PCR System. Expression relative to the endogenous gene and control group was calculated using the 2 −∆∆Ct method. Pairs of samples were compared using two-tailed t tests ( α = 0.05), applying Welch’s correction when necessary. The statistical differences were estimated by the Student’s t tests ( p < 0.05) on normalized data. Uncropped agarose gels are shown in Supplementary Figures 13 and 16 . Western blotting For total protein extraction, HeLa and human myoblast cells were sonicated while mouse muscles (gastrocnemius and quadriceps) were homogenized in RIPA buffer (150 mM NaCl, 1.0% IGEPAL, 0.5% sodium deoxycholate, 0.1% SDS, 50 mM Tris–HCl, pH 8.0) supplemented with protease and phosphatase inhibitor cocktails (Roche Applied Science). Total proteins were quantified with a BCA protein assay kit (Pierce) using bovine serum albumin as a standard concentration range. For the immunodetection assay, 20 μg of samples were denatured for 5 min at 100 °C, electrophoresed on 12% SDS-PAGE gels, transferred onto 0.45 µm nitrocellulose membranes (GE Healthcare), and blocked with 5% non-fat dried milk in PBS-T (8 mM Na 2 HPO 4 , 150 mM NaCl, 2 mM KH 2 PO 4 , 3 mM KCl, 0.05% Tween 20, pH 7.4). For HeLa cells, human myoblast, and murine samples, membranes were incubated overnight at 4 °C either with primary mouse anti-MBNL1 (1:1000, ab77017, Abcam) or mouse anti-CUG-BP1 (1:200, clone 3B1, Santa Cruz) antibodies. To detect MBNL2, mouse anti-MBNL2 (1:100, clone MB2a, Developmental Studies Hybridoma Bank) was used for human myoblast and mouse samples while rabbit anti-MBNL2 (1:1000, ab105331, Abcam) antibody was used for HeLa cells. All primary antibodies were detected using horseradish peroxidase (HRP)-conjugated anti-mouse-IgG secondary antibody (1 h, 1:5000, Sigma-Aldrich), except for the MBNL2 antibody in HeLa cell samples, which required a HRP-conjugated anti-rabbit-IgG secondary antibody (1 h, 1:5000, Sigma-Aldrich). Loading controls were the anti-β-ACTIN antibody (1 h, 1:5000, clone AC-15, Sigma-Aldrich) for cell samples and anti-Gapdh (1 h, 1:5000, clone G-9, Santa Cruz) for mouse samples, followed by HRP-conjugated anti-mouse-IgG secondary antibody (1 h, 1:5000, Sigma-Aldrich). Immunoreactive bands were detected using an enhanced chemiluminescence Western Blotting Substrate (Pierce) and images were acquired with an ImageQuant LAS 4000 (GE Healthcare). Quantification was performed using ImageJ software (NIH), and statistical differences were estimated using Student’s t test ( p < 0.05) on normalized data. Uncropped westerns are shown in Supplementary Figures 13 , 14 , and 15 . Luciferase reporter assay The activity of Gaussian luciferase (GLuc) and alkaline phosphatase (SEAP) were measured by quantifying the luminescence present in conditioned medium using the secreted-pair dual luminescence kit (GeneCopoeia) according to the manufacturer’s protocols. Gaussian luciferase activity was normalized to alkaline phosphatase activity (GLuc/SEAP). The values of the luciferase activity were determined using a Tecan Infinite M200 PRO plate reader (Life Sciences). Statistical differences in the data were estimated using Student’s t test ( p < 0.05) on normalized data. Cell proliferation assay Cells were seeded at 10 5 cells per ml in 96-well plates and transfected with antagomiRs, as previously explained; 96 h post-transfection, cell proliferation was measured using the CellTiter 96® AQueous Non-Radioactive Cell Proliferation Assay (Promega) following the manufacturer’s instructions. The TC 10 and dose–response inhibition curves were calculated using non-linear least squares regression, and absorbance levels were determined using a Tecan Infinite M200 PRO plate reader (Life Sciences). 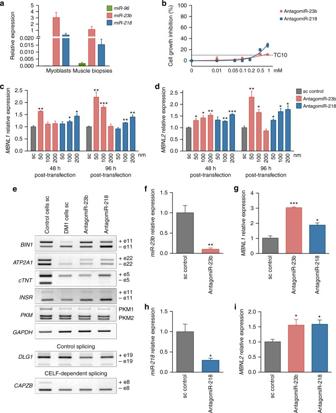Fig. 3 AntagomiR-23b and -218 stabilizeMBNLtranscripts and rescue alternative splicing defects in DM1 myoblasts.aReal-time PCR quantification ofmiR-96,miR-23b, andmiR-218expression in myoblasts and muscle biopsies from DM1 patients.U1andU6snRNAs were used as reference genes.bCell growth inhibition assay by MTS method. Human normal myoblasts were transfected with increasing concentrations of antagomiRs againstmiR-23bandmiR-218(n= 4). TC10 was obtained using the least squares non-linear regression model.c,dqRT-PCR quantification ofMBNL1(c) andMBNL2(d) expression relative toGAPDHandACTBgenes in human DM1 myoblasts transfected with the indicated antagomiRs or scrambled control antagomiR (sc).eSemiquantitative RT-PCR analyses of splicing events altered inBIN1(exon 11),ATP2A1(exon 22),cTNT(exon 5),INR(exon 11), andPKMisoforms in DM1 cells.GAPDHwas used as internal control. Inclusion ofDLG1exon 9, which is not altered in DM1, andCAPZBexon 8, which is CELF1-dependent, were used as additional controls.f,hmiRNA real-time PCR determination of availablemiR-23b(f) ormiR-218(h) in DM1 myoblasts 96 h after transfection with 50 nM of antagomiR-23b or 200 nM of antagomiR-218.U1andU6snRNAs were used as reference genes infandh.g,iqRT-PCR analyses ofMBNL1(g) andMBNL2(i) expression relative toGAPDHandACTBgenes in human myoblasts 96 h after transfection with 50 nM of antagomiR-23b or 200 nM of antagomiR-218. (n= 3). Data are mean ± SEM. *p< 0.05, **p< 0.01, ***p< 0.001 according to Student’sttest Immunofluorescence methods For MBNL1 and MBNL2, myoblasts were fixed with 4% PFA for 15 min at room temperature (RT) followed by several washes in 1× PBS. Cells were then permeabilized with PBS-T (0.3% Triton-X in PBS) and blocked (PBS-T, 0.5% BSA, 1% donkey serum) for 30 min at RT, and incubated either with primary antibody mouse anti-MBNL1 (1:200, ab77017, Abcam) or rabbit anti-MBNL2 (1:200, ab105331, Abcam) at 4 ° C overnight. After several PBS-T washes, the cells were incubated for 1 h with a biotin-conjugated secondary antibody, and anti-mouse-IgG (1:200, Sigma-Aldrich) to detect anti-MBNL1 or anti-rabbit-IgG (1:200, Sigma-Aldrich) to detect anti-MBNL2. The fluorescence signal was amplified with an Elite ABC kit (VECTASTAIN) for 30 min at RT, followed by PBS-T washes and incubation with either streptavidin-FITC (1:200, Vector) to detect anti-MBNL1 or streptavidin-Texas Red (1:200, Vector) to detect anti-MBNL2, for 45 min at RT. After several washes with PBS, the cells were mounted with VECTASHIELD® mounting medium containing DAPI (Vector) to detect the nuclei. The Cy3 moiety was synthetically attached to the 5′ end of the oligonucleotide to visualize the distribution of the compound. Frozen sections (10 μm) of mouse tissues including heart, brain, gastrocnemius, and quadriceps were immunostained using anti-Cy3 antibody (1:50, Santa Cruz) followed by a secondary goat biotin-conjugated anti-mouse-IgG (1:200, Sigma-Aldrich). Cy3‐labeled antagomiRs were directly detectable under a fluorescence microscope in myoblast cells. In all cases, the nuclei were stained with DAPI. Images of myoblast cells were taken on an Olympus FluoView FV100 confocal microscope and images of human myoblast and mouse tissues containing Cy3-antagomiR were obtained using a Leica DM4000 B LED fluorescence microscope. 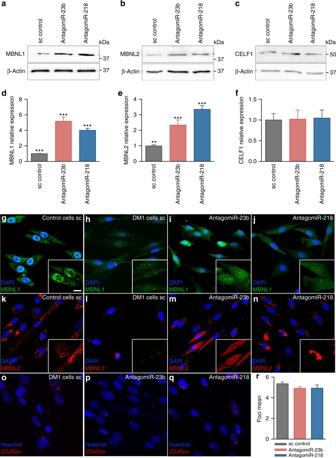Fig. 4 Increase of MBNL1 and MBNL2 upon silencing ofmiR-23bormiR-218in human myoblast.a–fWestern blot quantification of MBNL1 (a,d), MBNL2 (b,e), and CELF1 (c,f) expression levels in DM1 human myoblast 96 h after transfection with 50 nM of antagomiR-23b, 200 nM of antagomiR-218 or a scrambled control antagomiR (sc). β-ACTIN expression was used as endogenous control (n= 3). Data are mean ± SEM. **p< 0.01, ***p< 0.001 in Student’sttest.g–nRepresentative confocal images of MBNL1 (green) and MBNL2 (red) staining in healthy controls (control cells) and DM1 human myoblast 96 h after transfection with antagomiRs againstmiR-23b(50 nM) ormiR-218(200 nM) and a scrambled control antagomiR (DM1 cells). Nuclei were counterstained with DAPI (blue). In DM1 cells, endogenous MBNL1 (h) and MBNL2 (l) were in nuclear aggregates (green and red puncta) and the total amount of both was reduced compared to control cells (g) and (k), respectively. In contrast, DM1 cells treated with antagomiRs againstmiR-23bormiR-218showed a robust increase in cytoplasmic and nuclear MBNL1 (i,j) and MBNL2 (m,n) levels compared to DM1 cells.b–qRepresentative fluorescence of FISH images showing (CUG)n RNA foci (red) in DM1 human fibroblasts transfected with antagomiRs againstmiR-23b(50 nM) ormiR-218(200 nM) and a scrambled control antagomiR. Nuclei were counterstained with Hoechst (blue). AntagomiRs did not significant change the number of ribonuclear foci in DM1 fibroblasts (r). Scale bar = 20 μm In all cases, the images were taken at a 40× magnification and processed with Adobe Photoshop software (Adobe System Inc.). Fluorescent in situ hybridization Fibroblasts were aliquoted into 8-well Cell Culture Slide (3 × 10 5 cells per well) and transfected with the antagomiRs. In situ detection was performed as previously described [65] . Images were taken and analyzed using an IN Cell Analyzer 2200 Imaging System (GE Healthcare). Electromyography studies Electromyography was performed before the treatment, at the halfway point and at the time of sacrifice under general anesthesia, as previously described [32] . Briefly, five needle insertions were performed in each quadriceps muscle of both hind limbs, and myotonic discharges were graded on a five-point scale: 0, no myotonia; 1, occasional myotonic discharge in ≤50% of the needle insertions; 2, myotonic discharge in >50% of the insertions; 3, myotonic discharge in nearly all of the insertions; and 4, myotonic discharge in all insertions. Muscle histology Frozen 15 μm-sections of mouse gastrocnemius and quadriceps muscles were stained with haematoxylin eosin (H&E) and mounted with VECTASHIELD® mounting medium (Vector) according to standard procedures. Images were taken at a 100× magnification with a Leica DM2500 microscope. The percentage of fibers containing central nuclei was quantified in a total of 500 fibers in each mouse. Forelimb grip strength test The forelimb grip strength was measured with a Grip Strength Meter (BIO-GS3; Bioseb, USA). The peak pull force (measured in grams) was recorded on a digital force transducer when the mouse grasped the bar. The gauge of force transducer was reset to 0 g after each measurement. Tension was recorded by the gauge at the time the mouse released its forepaws from the bar. We performed three consecutive measurements at 30 s intervals. 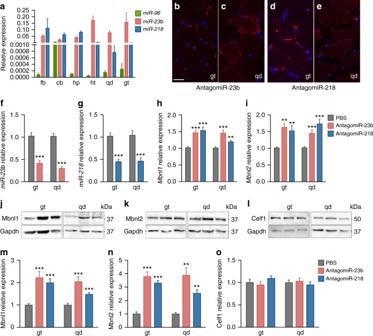Fig. 5 Subcutaneous injection of antagomiR-23b or antagomiR-218 in HSALRmice reduced target miRNA levels and increased Mbnl1 and Mbnl2 without affecting levels of Celf1.aqPCR quantification ofmiR-96,miR-23b, andmiR-218expression levels in forebrain (fb), cerebellum (cb), hippocampus (hp), heart (ht), and quadriceps (qd) and gastrocnemius (gt) muscles (n= 3). Average expression levels ofU1andU6were used for normalization.b–eImmunodetection of Cy3-labeled antagomiRs in gastrocnemius (b,d) and quadriceps (c,e) cryosections of HSALRtreated mice (n= 1). Myonuclei were counterstained with DAPI (blue). Scale bar = 50 μm.f–gQuantification ofmiR-23bandmiR-218in gt and qd muscles of untreated mice (PBS, gray bars) or treated with antagomiR-23b (pink bars) or antagomiR-218 (blue bars). Relative values (to average ofU1andU6expression) were further normalized to the levels in untreated mice.h, iReal-time PCR quantification ofMbnl1andMbnl2transcript levels in gt and qd muscles. Expression levels relative to the endogenousGapdhwere normalized to the levels in untreated mice.j–oWestern blotting analysis of Mbnl1 (j,m), Mbnl2 (k,n), and Celf1 (l,o) proteins in mouse gt and qd muscles. Representative blots used for quantification in (m–o) are shown in (j–l). The data were analyzed by unpaired Student’sttest compared to untreated HSALRmice. Data are mean ± SEM. *p< 0.05, **p< 0.01, ***p< 0.001; HSALRPBS (n= 10 inf–o), HSALRantagomiR-23b (n= 9, inf–o). HSALRantagomiR-218 (n= 9, inf–o) 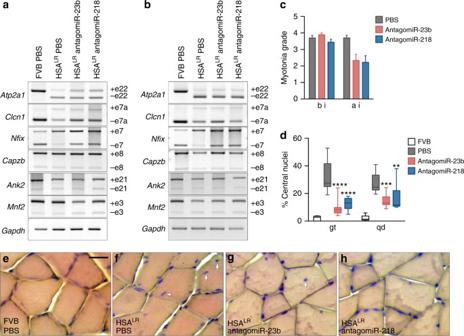Fig. 6 Systemic delivery of antagomiRs improved missplicing of Mbnl-dependent transcripts, myotonia, and muscle histopathology in HSALRmice.a,bRT-PCR analyses of the splicing ofAtp2a1exon 22,Clcn1exon 7a,Nfixexon 7,Capzbexon 8,Ank2exon 21, andMnf2exon 3 in gastrocnemius (gt) (a) and quadriceps (qd) (b) muscles.Gadphvalues were used for normalization in the quantification of the exon inclusion in Supplementary Figs.9and11.cElectromyographic myotonia grade in antagomiR (pink and blue bars) or PBS-treated (gray bars) HSALRmice before (bi) and 4 days after injection (ai). Data are mean ± SEM.dQuantification of the percentage of muscle fibers with central nuclei in gt and qd muscles of control FVB (white bar), and PBS (gray bar) or antagomiR-treated (pink and blue bars) HSALRmice.e–hRepresentative hematoxylin and eosin staining of gt muscles from all four groups of mice. Arrows point to examples of centrally located nuclei in muscle fibers. Scale bar = 50 μm. The data were analyzed by unpaired Student’sttest compared to untreated HSALRmice. Data are media ± SEM. *p< 0.05; FVB (n= 3), HSALRPBS (n= 5), HSALRantagomiR-23b (n= 4) and HSALRantagomiR-218 (n= 4) 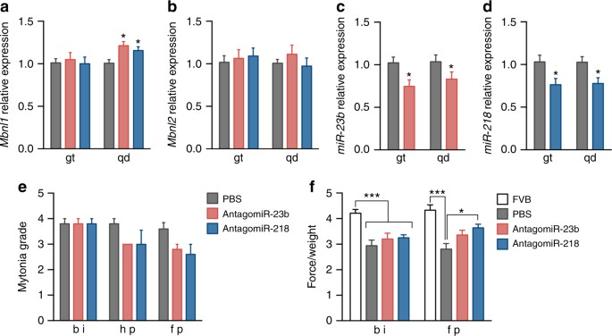Fig. 7 Muscle function is improved in HSALRmice 6 weeks after injection of antagomiRs.a,bqRT-PCR quantification ofMbnl1andMbnl2transcript levels in gt and qd muscles of untreated mice (PBS, gray bars) or treated with antagomiR-23b (pink bars) or antagomiR-218 (blue bars).c,dReal-time PCR quantification ofmiR-23bandmiR-218.eElectromyographic myotonia grade in antagomiR (pink and blue bars) or PBS-treated (gray bars) HSALRmice before (bi), in the halfway-point (hp) and 6 weeks after injection (final point, fp).fForelimb grip strength of mice treated with antagomiRs measured before injection (bi) and 6 weeks after injection (fp). The grip force was normalized with the body weight of each mouse. The data were analyzed by unpaired Student’sttest compared to HSALRmice treated with the vehicle PBS. Data are mean ± SEM. *p< 0.05, ***p< 0.001; FVB (n= 5), HSALRPBS (n= 6), HSALRantagomiR-23b (n= 5) and HSALRantagomiR-218 (n= 5) The bodyweight measurement was performed in parallel. The final value is obtained by dividing the average value of the grip force with the body weight of each mouse. Data availability All relevant data are available within the manuscript and its supplementary information or from the authors upon reasonable request. Please contact Rubén Artero (Ruben.artero@uv.es) for any inquire.